Crossreactivity to vinculin and microbes provides a molecular basis for HLA-based protection against rheumatoid arthritis The HLA locus is the strongest risk factor for anti-citrullinated protein antibody (ACPA) + rheumatoid arthritis (RA). Despite considerable efforts in the last 35 years, this association is poorly understood. Here we identify (citrullinated) vinculin, present in the joints of ACPA + RA patients, as an autoantigen targeted by ACPA and CD4 + T cells. These T cells recognize an epitope with the core sequence DERAA, which is also found in many microbes and in protective HLA-DRB1*13 molecules, presented by predisposing HLA-DQ molecules. Moreover, these T cells crossreact with vinculin-derived and microbial-derived DERAA epitopes. Intriguingly, DERAA-directed T cells are not detected in HLA-DRB1*13 + donors, indicating that the DERAA epitope from HLA-DRB1*13 mediates (thymic) tolerance in these donors and explaining the protective effects associated with HLA-DRB1*13. Together our data indicate the involvement of pathogen-induced DERAA-directed T cells in the HLA–RA association and provide a molecular basis for the contribution of protective/predisposing HLA alleles. Rheumatoid arthritis (RA) is a chronic autoimmune disease affecting synovial joints that can lead to severe disability. Pivotal pathophysiological insight has been obtained by the identification of anti-citrullinated protein antibodies (ACPA) [1] , [2] . These autoantibodies target proteins that have undergone a post-translational conversion of arginine to citrulline, catalysed by peptidylarginine deiminases (PAD enzymes) [3] . ACPA are highly specific for RA, enriched in the joints of patients and can crossreact between citrullinated antigens that are expressed in the inflamed joints [4] , [5] , [6] , [7] , [8] . It is clear now that RA represents two main syndromes, ACPA + and ACPA − disease, each with distinct genetic and environmental risk factors and disease outcome [9] , [10] , [11] , [12] . Characteristics of ACPA (for example, isotype usage and epitope spreading) indicate the involvement of CD4 + T cell help in shaping the ACPA response [13] . The most important genetic risk factor for ACPA + RA is the HLA class II locus and risk is confined to a region with genes encoding for the beta chain of HLA-DR and the alpha and beta chain of HLA-DQ that are in tight linkage disequilibrium (LD) and inherited in haplotypes [14] , [15] . An understanding of the HLA class II association and the relative contribution of the HLA-DR and HLA-DQ locus has been lacking for the last 35 years. Next to the association of the predisposing alleles to ACPA + RA, other HLA molecules are associated with protection. These protective HLA alleles, mainly HLA-DRB1*13, carry the five amino-acid sequence DERAA at positions 70–74 of the beta chain and protect also in the presence of predisposing alleles [16] , [17] . Intriguingly, protection by these alleles is transferred from mother to child, supporting an active protective role of these alleles, possibly via microchimeric cells influencing thymic selection of CD4 + T cells, and indicating a dominant role of HLA-DRB1*13 in disease protection [18] . HLA-derived peptides are a dominant peptide source presented by HLA class II molecules. We therefore proposed that the protective effect of HLA-DRB1*13 is explained by presentation of an HLA-DRB1*13-derived peptide in the context of other (predisposing) HLA class II molecules [19] , [20] , [21] . It was previously shown that the degradation of HLA-DRB1*13 can result in the presentation of a peptide with the core sequence DERAA by other HLA class II molecules to CD4 + T cells [22] . This could allow for the negative selection of such ‘DERAA-directed’ CD4 + thymocytes. Interestingly, the DERAA sequence is also found in many microbes and in the self-protein vinculin. Vinculin is expressed in the synovium and was recently shown to be citrullinated in the synovial fluid of an RA patient [4] , [23] . Likewise, T cells directed to vinculin are found under certain infectious conditions, indicating that T cell tolerance to vinculin is not absolute [24] , [25] . Molecular mimicry of self-proteins with pathogenic proteins was proposed as an important mechanism to break T cell tolerance [26] , [27] . Therefore, we postulate that on priming of DERAA-directed T cells by microbes expressing DERAA-containing proteins, T cells crossreactive to vinculin would be able to provide help to B cells reactive to citrullinated vinculin. This would ultimately result in the production of ACPA. In HLA-DRB1*13-positive donors, these T cells are conceivably deleted, leading to protection against ACPA + disease. Here we show that citrullinated vinculin is novel autoantigen for ACPA antibodies. In addition, we demonstrate the presence of a T cell population in HLA-DRB1*13-negative donors that specifically recognize a DERAA-containing vinculin epitope and that crossreact with DERAA sequences derived from pathogens. Citrullinated vinculin is a novel target for ACPA We speculate that the protective effects of HLA-DRB1*13 on the development of ACPA + RA are related to a T cell response reactive to a sequence that is commonly present in the HLA-DRB1*13 molecule, microorganisms and self-proteins that are targeted by ACPA. Indeed, a 5-amino-acid long HLA-DRB1*13-derived sequence (DERAA) is present in many microorganisms and a few self-proteins. Of these self-proteins, the citrullinated protein vinculin attracted our attention. Therefore, we first analysed whether citrullinated vinculin is recognized by ACPA. To this end, we citrullinated vinculin in vitro with PAD enzymes and tested both native and citrullinated vinculin for recognition with serum of an ACPA + RA patient. We observed citrulline-specific recognition of vinculin by serum of an ACPA + RA patient, but not with an ACPA − patient ( Fig. 1a ). We further confirmed that citrullinated vinculin is a target of ACPA using an ACPA monoclonal antibody ( Fig. 1b ) [28] . 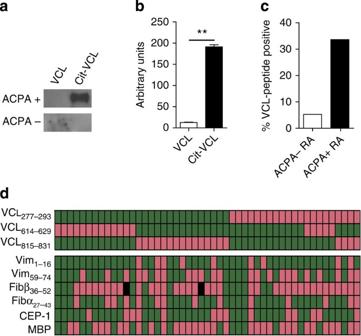Figure 1: Citrullinated vinculin is a novel autoantigen targeted by ACPA. (a) Western blot (Supplementary Fig. 22) of native and citrullinated vinculin protein, stained with the serum of an ACPA+or an ACPA−RA patient. (b) Enzyme-linked immunosorbent assay (ELISA) of vinculin- or citrullinated vinculin protein-coated plates stained with ACPA monoclonal antibody anti-citFib1.1. Two-sided statistical analysis was performed using a Student’st-test with ** indicatingP<0.001. Error bar is s.e.m. (c) ELISA of citrullinated vinculin peptides VCL-CIT285277–293, VCL-CIT622614–651, VCL-CIT823815–831in serum of anti-CCP2+(n=140) versus anti-CCP2−(n=38) RA patients. Plot depicts the percentage of patient sera positive for one or more citrullinated vinculin peptides. (d) Heat map depicting all patients positive for one or more citrullinated vinculin epitopes (n=49) and their serum reactivity towards different citrullinated epitopes derived from vimentin, fibrinogen and alpha-enolase. Red, positive; green, negative; black, undetermined. Error bars are s.e.m. Figure 1: Citrullinated vinculin is a novel autoantigen targeted by ACPA. ( a ) Western blot ( Supplementary Fig. 22 ) of native and citrullinated vinculin protein, stained with the serum of an ACPA + or an ACPA − RA patient. ( b ) Enzyme-linked immunosorbent assay (ELISA) of vinculin- or citrullinated vinculin protein-coated plates stained with ACPA monoclonal antibody anti-citFib1.1. Two-sided statistical analysis was performed using a Student’s t -test with ** indicating P <0.001. Error bar is s.e.m. ( c ) ELISA of citrullinated vinculin peptides VCL-CIT285 277–293 , VCL-CIT622 614–651 , VCL-CIT823 815–831 in serum of anti-CCP2 + ( n =140) versus anti-CCP2 − ( n =38) RA patients. Plot depicts the percentage of patient sera positive for one or more citrullinated vinculin peptides. ( d ) Heat map depicting all patients positive for one or more citrullinated vinculin epitopes ( n =49) and their serum reactivity towards different citrullinated epitopes derived from vimentin, fibrinogen and alpha-enolase. Red, positive; green, negative; black, undetermined. Error bars are s.e.m. Full size image Recently, several reports showed the presence of citrullinated vinculin in the synovial fluid of ACPA + RA patients. In addition, three sites of in vivo citrullination on this protein were identified: Arg285, Arg622 and Arg823 (refs 4 , 23 ). When we studied antibody responses to these citrullination sites, we could show recognition by 34% of tested sera from ACPA + RA patients versus 5% of sera from ACPA − patients ( Fig. 1c ). Sera of ACPA + RA patients are highly (cross-)reactive towards multiple citrullinated antigens. Indeed, when we quantified responses to citrullinated alpha-enolase, fibrinogen, vimentin and myelin basic protein in patient sera that react to citrullinated vinculin peptides, we could readily demonstrate additional reactivities indicating that ACPA are not exclusively directed against citrullinated vinculin as expected ( Fig. 1d ). Together these data show that citrullinated vinculin is a self-protein recognized by RA autoantibodies in a citrulline-dependent fashion. Vinculin is recognized by T cells from HLA-DRB1*13 negative donors We next wished to determine whether the DERAA sequence from vinculin is recognized by human CD4 + T cells. To this end, peripheral blood mononuclear cells (PBMCs) were stimulated with a 15-mer vinculin-peptide (VCL 622–636 , REEVFDERAANFENH) (VCL-DERAA) for 24 h. We observed a clear reactivity towards this epitope as determined in an interferon-γ (IFN-γ)-ELISPOT-assay ( Supplementary Fig. 1 ). HLA-DRB1*13, especially HLA-DRB1*13:01, is strongly associated with protection against ACPA + RA [17] . We hypothesize that HLA-DRB1*13 protects against ACPA + disease by affecting the generation of DERAA-directed T cells. Therefore, we stratified donors for HLA-DRB1*13:01 status. We observed a striking difference in IFN-γ-producing cells depending on HLA-DRB1*13:01-status. The lack of reactivity in HLA-DRB1*13:01-positive donors was not due to a hampered ability of such donors to respond to T cell antigens as we observed strong response to microbial antigens in both HLA-DRB1*13:01 carriers and non-carriers when stimulated with recall antigens ( Fig. 2a ). We further confirmed this finding in PBMCs stimulated for 4 days ( Supplementary Fig. 2 ). The differential ability of HLA-DRB1*13:01-positive donors to respond to VCL-DERAA is most likely not due to a general deficiency to present the VCL-DERAA epitope as these donors were heterozygous and thus expressed other HLA molecules that could potentially present VCL-DERAA. Nonetheless, to further confirm that HLA-DRB1*13:01 affects the ability to generate VCL-DERAA-directed T cell responses, we repeated the experiments in a set-up stratified for HLA using PBMCs from HLA-DRB1*04-, HLA-DRB1*13:01- and HLA-DRB1*04/*13:01 heterozygous donors. A significant reduction in IFN-γ-producing cells was observed in both HLA-DRB1*13:01 carriers and DRB1*04/*13:01 heterozygous donors as compared with HLA-DRB1*04 carriers. Again, no difference was observed for recall antigens ( Fig. 2b ). These data indicate that the lack of detecting VCL-DERAA-directed T cells is not explained by the inability of HLA-DRB1*13 molecules to present VCL-DERAA, but rather the result of a dominant effect associated with the presence of HLA-DRB1*13. 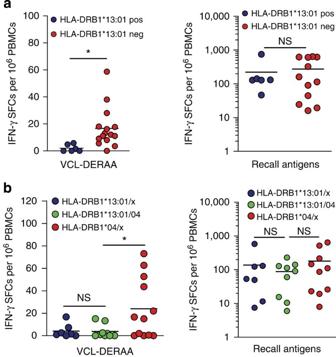Figure 2: Citrullinated vinculin is a novel autoantigen targeted by CD4+T cells in HLA-DRB1*13-negative donors. (a) IFN-γ ELISPOT of PBMCs from healthy individuals stimulated for 24 h with VCL-DERAA peptide REEVFDERAANFENH (n=21) or with a mix of recall antigens (tetanus, tuberculin, candida,n=18). Donors were stratified based on HLA-DRB1*13:01 status. (b) IFN-γ ELISPOT of PBMCs of HLA-DRB1*13:01 carriers (n=7), HLA-DRB1*04 carriers (n=12) and HLA-DRB1*13:01/DRB1*04 donors (n=9), stimulated for 24 h with VCL-DERAA peptide or with a mix of recall antigens. Each dot represents a unique donor. Two-sided statistical analyses of ELISPOT data were performed using a Mann–WhitneyU-test with * indicatingP<0.05. Neg, negative; NS, not significant; Pos, positive. Figure 2: Citrullinated vinculin is a novel autoantigen targeted by CD4 + T cells in HLA-DRB1*13-negative donors. ( a ) IFN-γ ELISPOT of PBMCs from healthy individuals stimulated for 24 h with VCL-DERAA peptide REEVFDERAANFENH ( n =21) or with a mix of recall antigens (tetanus, tuberculin, candida, n =18). Donors were stratified based on HLA-DRB1*13:01 status. ( b ) IFN-γ ELISPOT of PBMCs of HLA-DRB1*13:01 carriers ( n =7), HLA-DRB1*04 carriers ( n =12) and HLA-DRB1*13:01/DRB1*04 donors ( n =9), stimulated for 24 h with VCL-DERAA peptide or with a mix of recall antigens. Each dot represents a unique donor. Two-sided statistical analyses of ELISPOT data were performed using a Mann–Whitney U -test with * indicating P <0.05. Neg, negative; NS, not significant; Pos, positive. Full size image Thus, vinculin is an autoantigen recognized by circulating VCL-DERAA-directed CD4 + T cells. In HLA-DRB1*13:01 carriers these T cells are absent. This effect, like the protective effects of HLA-DRB1*13:01 on the development of ACPA + RA, was present in a dominant fashion, consistent with the notion that HLA-DRB1*13 affects the generation of DERAA-directed T cells, possibly during thymic selection. Presentation of Vinculin-DERAA by RA-predisposing HLA-DQ molecules HLA-DRB1 alleles predisposing to ACPA + RA in the Caucasian population are collectively called HLA shared epitope (SE) alleles [14] , [15] , [29] . The most common HLA-SE alleles are HLA-DRB1*04:01 and HLA-DRB1*01:01. Using HLA-DR-binding assays, we examined the ability of VCL-DERAA to bind to these HLA molecules, but we could not detect any binding of VCL-DERAA to these alleles ( Table 1 , Supplementary Fig. 3a,b ). The HLA class II region is known for its strong LD. Genes that encode for the HLA-DR-beta chains are inherited in haplotypes with genes that encode for the alpha and beta chain of HLA-DQ. The predisposing HLA-SE alleles are in tight LD with HLA-DQ5 (DQA1*01;DQB1*05:01), HLA-DQ7.3 (DQA1*03:02;DQB1*03:01) and HLA-DQ8 (DQA1*03:01;DQB1*03:02) ( Fig. 3a,b ). In Fig. 3b , the distribution of HLA-DQ molecules in SE+ healthy donors is depicted, showing that these donors are HLA-DQ5-, HLA-DQ7.3- or HLA-DQ8 positive. We therefore next studied the binding of VCL-DERAA to these HLA-DQ alleles and observed binding of the VCL-DERAA peptide to HLA-DQ5, DQ7.3 and DQ8 ( Table 1 , Supplementary Fig. 3c–e ). These data indicate that VCL-DERAA can be presented by HLA-DQ molecules in LD with predisposing HLA-SE alleles. Table 1 Presentation to vinculin-DERAA-directed T cells is restricted to RA-predisposing HLA-DQ molecules. 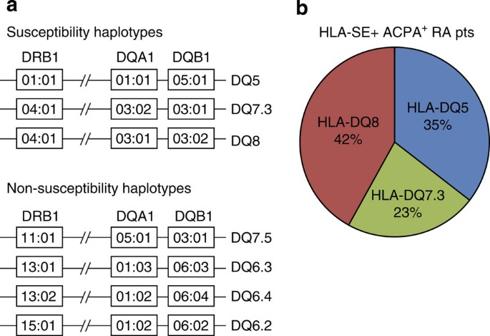Figure 3: Presentation to vinculin-DERAA-directed T cells is restricted to RA-predisposing HLA-DQ molecules. (a) Schematic representation of the LD between the HLA-DRB1, HLA-DQA1 and HLA-DQB1 gene in studied haplotypes associated or not associated with susceptibility to ACPA+RA. (b) Distribution of HLA-DQ molecules in ACPA+RA patients positive for HLA-DR SE alleles (n=31). Full size table Figure 3: Presentation to vinculin-DERAA-directed T cells is restricted to RA-predisposing HLA-DQ molecules. ( a ) Schematic representation of the LD between the HLA-DRB1, HLA-DQA1 and HLA-DQB1 gene in studied haplotypes associated or not associated with susceptibility to ACPA + RA. ( b ) Distribution of HLA-DQ molecules in ACPA + RA patients positive for HLA-DR SE alleles ( n =31). Full size image To obtain an indication whether the VCL-DERAA can be presented by more HLA molecules, we also studied the ability of additional HLA-DR and HLA-DQ molecules encoded by HLA haplotypes that protect or have no influence on the development of ACPA + RA. We could not detect binding of VCL-DERAA to these HLA class II alleles ( Table 1 , Supplementary Fig. 3f–k ). Likewise, using an IFN-gamma ELISPOT, VCL-DERAA-directed T cells were absent in donors negative for predisposing HLA-DQ molecules ( Supplementary Fig. 4 ). These data indicate that HLA-DQ molecules that predispose to ACPA + disease present the VCL-DERAA peptide, whereas the analysed HLA-DQ and HLA-DR molecules not associated with disease do not present VCL-DERAA. HLA-DQ-restricted recognition of VCL-DERAA by T cells To further confirm the presence of VCL-DERAA-directed T cells and their HLA-restriction, we isolated CD4 + T cell clone JPT57, which was specific for VCL-DERAA. As shown in Supplementary Fig. 5 , this clone proliferated readily and produced large amounts of IFN-γ when stimulated with the VCL-DERAA peptide. When cultured with B cells from ACPA + RA patients pulsed with the VCL-DERAA epitope, the clone not only upregulated CD40L, but also enhanced the production of ACPA in culture, indicating that such T cells have a phenotype compatible with the ability to provide ‘help’ to ACPA-producing B cells ( Supplementary Fig. 6 ). To further confirm that HLA-DQ molecules present the VCL-DERAA peptide, we stimulated the clone with VCL-DERAA-pulsed HLA-typed antigen-presenting cells preincubated with HLA class II blocking antibodies ( Supplementary Fig. 7 ). In concordance with the binding studies, anti-HLA-DQ antibodies abrogated T cell recognition. Interestingly, we observed that JPT57 can recognize VCL-DERAA, presented by both HLA-DQ7.3 and HLA-DQ8 suggesting that this epitope is presented in a similar binding register by these HLA molecules ( Supplementary Fig. 8 ). Together HLA class II presentation and T cell recognition of VCL-DERAA was restricted to HLA-DQ molecules that are associated with RA susceptibility. Identification of microbe-specific T cells targeting DERAA epitopes We next investigated the presence of the DERAA sequence in microorganisms. A Blast search showed that DERAA is found in 66% of bacteria and 4% of viruses ( Fig. 4a ). This large number represents a major challenge to identify potential ‘crossreactive microorganisms’. To select for relevant microorganisms, we restricted the search to those microorganisms that can cause disease or symptoms in humans and are present in the western world. This approach left us with 219 candidate sequences. We then synthesized eight DERAA-containing peptides from common recall microbes including several bacteria ( P. acnes , S enteritidis , B. pertussis , S. aureus ) and viruses (measles virus, influenza A and human herpesvirus 7). Interestingly, all of these peptides were presented by HLA-DQ7.3 and DQ8 molecules showing that these HLA molecules can efficiently accommodate both the VCL-DERAA epitope as well as microbe-derived DERAA epitopes ( Fig. 4b ). 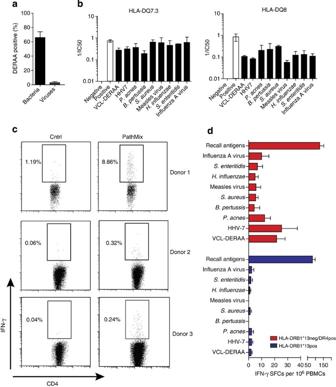Figure 4: Identification of pathogen-specific T cells targeting DERAA epitopes in HLA-DRB1*13 negative donors. (a) Frequency of bacteria or viruses positive for a DERAA-containing protein as identified using the NCBI BLAST. List of all bacteria or viruses in blast database was generated and for three random sets of 50 bacteria/viruses a blast search for DERAA was performed. Error bars indicate the s.d. between the three analysed sets. (b) Competitive binding of pathogen-derived DERAA epitopes to HLA-DQ7.3 or HLA-DQ8. Binding experiments were performed at least three times and plots show pooled experiments, the error bars show the variation between the different experiments. (c) Flow cytometry staining of PathMix-directed T cell lines restimulated with PathMix pulsed or unpulsed antigen-presenting cells. Plots are gated on CD14neg/CD4pos/CD25pos T cells. (d) ELISPOT of PBMCs of healthy individuals of HLA-DRB1*13:01 donors (n=5) and HLA-DQ7.3/DQ8 donors (n=8) stimulated for 24 h with DERAA-containing peptides and recall antigens. Error bars indicate the variation between different donors. Error bars are s.e.m. Figure 4: Identification of pathogen-specific T cells targeting DERAA epitopes in HLA-DRB1*13 negative donors. ( a ) Frequency of bacteria or viruses positive for a DERAA-containing protein as identified using the NCBI BLAST. List of all bacteria or viruses in blast database was generated and for three random sets of 50 bacteria/viruses a blast search for DERAA was performed. Error bars indicate the s.d. between the three analysed sets. ( b ) Competitive binding of pathogen-derived DERAA epitopes to HLA-DQ7.3 or HLA-DQ8. Binding experiments were performed at least three times and plots show pooled experiments, the error bars show the variation between the different experiments. ( c ) Flow cytometry staining of PathMix-directed T cell lines restimulated with PathMix pulsed or unpulsed antigen-presenting cells. Plots are gated on CD14neg/CD4pos/CD25pos T cells. ( d ) ELISPOT of PBMCs of healthy individuals of HLA-DRB1*13:01 donors ( n =5) and HLA-DQ7.3/DQ8 donors ( n =8) stimulated for 24 h with DERAA-containing peptides and recall antigens. Error bars indicate the variation between different donors. Error bars are s.e.m. Full size image To determine whether these microbial-derived epitopes are recognized by human T cells, we generated T cell lines by stimulating PBMCs from three healthy HLA-DQ8-positive donors for 7 days with a pool of the eight pathogen-derived peptides (PathMix). Next we determined the presence of PathMix-specific CD4 + IFN-γ-producing T cells. As shown in Fig. 4c , such T cells were readily detectable. Using limiting dilutions, we isolated T cell clone D2C18, further confirming the presence of ‘microbial-DERAA-directed’ T cells ( Supplementary Fig. 9 ). Next we also analysed the presence of ‘microbial-DERAA-directed’ T cells by ELISPOT directly ex vivo , allowing the analyses of more donors at higher throughput. Interestingly, PBMCs from HLA-DRB1*13:01 carriers displayed a significantly reduced reaction against these peptides, indicating that the presence of HLA-DRB1*13 also affects the formation of T cell responses against DERAA epitopes from microbes ( Fig. 4d ). Together these data indicate that HLA-DQ alleles associated with ACPA + RA efficiently present both VCL-DERAA and microbe-derived DERAA epitopes and that microbe-specific T cells directed to DERAA epitopes are readily detected. The presence of HLA-DRB1*13:01 affects the formation of these T cell responses. Predicting crossreactive microbes by modelling vinculin-DERAA presentation The data presented above demonstrate the presence of microbial- and VCL-DERAA-directed T cells, but do not show if a single T cell receptor (TCR) can react with both epitopes. To facilitate the search for possible ‘crossreactive’ DERAA epitopes out of all microbe-derived DERAA sequences, we first determined the binding register of VCL-DERAA using HLA class II-binding assays with amino (N)- and carboxyl (C)-terminally truncated and amino-acid-substituted VCL-DERAA peptides as detailed in the Supplementary Note and in Supplementary Figs 10–14 . Together these experiments support V FD E R AA N F (anchors in bold) as the core binding register for both HLA-DQ7.3 and HLA-DQ8. All-atom molecular dynamics (MD) simulations showed that residues Val625 (P1), Glu628 (P4) and Phe633 (P9) make numerous intermolecular polar and non-polar interactions in the respective pockets. In Fig. 5a–f , we highlight key intermolecular interactions between the VCL-DERAA epitope and the HLA-DQ8 molecule. A detailed discussion of the MD results and a quantitative assessment of the intermolecular interactions can be found in the supplementary data ( Supplementary Figs 15 and 16 , Supplementary Table 1 and Supplementary Note ). The MD simulations also indicated that the long protruding side chains of Glu623 (P-2) Glu624 (P-1), Phe626 (P2), Asp627 (P3), Arg629 (P5), Asn632 (P8), Glu634 (P10) and Asn635 (P11) are exposed and could potentially interact with crossreactive TCRs ( Fig. 5g ). Subsequently we also further confirmed the obtained model using a second type of molecular modelling: energy minimization, which further confirmed possible TCR-contact residues ( Supplementary Figs 17 and 18 ). 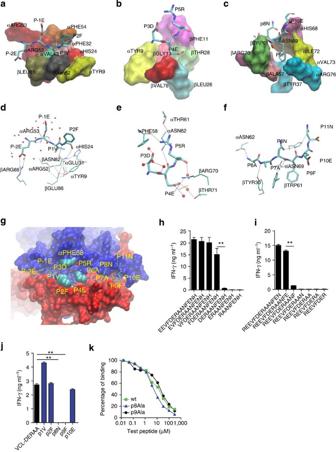Figure 5: Molecular modelling of HLA:VCL-DERAA complexes identifies critical TCR-contact residues. (a–c) Non-polar contacts between the VCL-DERAA peptide and HLA-DQ8 in pockets P1 (a), P4 (b) and P9 (c). Protein residues are depicted in a surface representation, in distinct colours. (d–f)Hydrogen bonds between the VCL-DERAA peptide and HLA-DQ8 in pockets P1 (d), P4 (e) and P9 (f). Peptide and protein groups are shown, respectively, in thick and thin licorice representation and water molecules as small spheres. Hydrogens are omitted, with the exception of the extra hydrogen in protonated αGlu31. (g) TCR view of the DQ8:VCL-DERAA complex. The peptide main chain is shown in licorice; domains α and β are shown in a surface representation, coloured, respectively, in blue and red. Side chains P-2E, P-1E, P2F, P3D, P5R, P8N, P10E and P11N are facing towards the TCR-binding site. The P2F and αPhe58 side chains and the non-polar moiety of P5R form a non-polar cluster, which faces towards the TCR-binding site; the average P2F ring–αPhe58 ring distance is∼8 Å. (h–j) IFN-γ ELISA on supernatant of T cell clone JPT57 stimulated with unpulsed HLA-DQ8-positive antigen-presenting cells and N-truncated (h), C-truncated (i) or alanine-substituted (j) VCL-DERAA peptides. (k) Competitive binding of the VCL-DERAA peptide, and alanine-substituted VCL-DERAA peptides to HLA-DQ8. Binding experiments were performed at least three times and plots show pooled experiments, the error bars show the variation between the different experiments. Experiments involving JPT57 were performed three times and show a representative experiment. Two-sided statistical analysis was performed using a Student’st-test with ** indicatingP<0.001. Error bars are s.e.m. Figure 5: Molecular modelling of HLA:VCL-DERAA complexes identifies critical TCR-contact residues. ( a – c ) Non-polar contacts between the VCL-DERAA peptide and HLA-DQ8 in pockets P1 ( a ), P4 ( b ) and P9 ( c ). Protein residues are depicted in a surface representation, in distinct colours. ( d – f) Hydrogen bonds between the VCL-DERAA peptide and HLA-DQ8 in pockets P1 ( d ), P4 ( e ) and P9 ( f ). Peptide and protein groups are shown, respectively, in thick and thin licorice representation and water molecules as small spheres. Hydrogens are omitted, with the exception of the extra hydrogen in protonated αGlu31. ( g ) TCR view of the DQ8:VCL-DERAA complex. The peptide main chain is shown in licorice; domains α and β are shown in a surface representation, coloured, respectively, in blue and red. Side chains P-2E, P-1E, P2F, P3D, P5R, P8N, P10E and P11N are facing towards the TCR-binding site. The P2F and αPhe58 side chains and the non-polar moiety of P5R form a non-polar cluster, which faces towards the TCR-binding site; the average P2F ring–αPhe58 ring distance is ∼ 8 Å. ( h – j ) IFN-γ ELISA on supernatant of T cell clone JPT57 stimulated with unpulsed HLA-DQ8-positive antigen-presenting cells and N-truncated ( h ), C-truncated ( i ) or alanine-substituted ( j ) VCL-DERAA peptides. ( k ) Competitive binding of the VCL-DERAA peptide, and alanine-substituted VCL-DERAA peptides to HLA-DQ8. Binding experiments were performed at least three times and plots show pooled experiments, the error bars show the variation between the different experiments. Experiments involving JPT57 were performed three times and show a representative experiment. Two-sided statistical analysis was performed using a Student’s t -test with ** indicating P <0.001. Error bars are s.e.m. Full size image To functionally confirm whether a TCR would indeed interact with (some of the) potential TCR-contact residues within the VCL-DERAA peptide, we next determined how the epitope is recognized by the VCL-DERAA-directed T cell clone JPT57. Phe626 (P2) interacts with the JPT57–TCR as its removal results in a large decrease in recognition without affecting HLA-DQ8 binding. ( Fig. 5h , Supplementary Fig. 12 ). C-terminal truncations resulted in a large decrease in T cell recognition after the removal of Glu634 (P10), showing that this residue is also important for JPT57–TCR interaction ( Fig. 5i ). Thus, the data obtained using the VCL-DERAA-directed T cell clone as a functional read-out, are in line with the HLA-binding and molecular modelling studies indicating the sequence V FD E R AA N F E (anchors in bold) as the minimal epitope required for activation of JPT57. Next we performed alanine substitutions within the minimal epitope to remove critical TCR-interacting residues. Substituting Asn632 (P8) and Phe633 (P9) dramatically impacted T cell recognition, without affecting the binding affinity of VCL-DERAA ( Fig. 5j,k ). Together these data indicate V FD E R AA N F (anchors in bold) as the most likely core binding register for HLA-DQ7.3 and HLA-DQ8 and Asn632 and Phe633 as important residues for JPT57–TCR recognition. TCR crossreactivity between vinculin and bacterial antigens Identifying microbes that crossreact with vinculin was challenging due to the large number of potential candidates. Therefore, we used the data presented above to determine if a single TCR can crossreact both to DERAA sequences from microbes and the self-protein vinculin. As we identified the Asn632 and Phe633 at P8 and P9, respectively, as important for JPT57–TCR interactions, we used the molecular modelling to predict which viral and bacterial epitopes are likely to bind to HLA-DQ8 and harbor P8Asn or P9Phe and are thus likely to crossreact with JPT57. From the 15 peptides identified ( Supplementary Table 2 ), three were able to activate JPT57 in a T cell stimulation assay at concentrations similar to those used for the vinculin peptide. These epitopes were derived from Campylobacter coli , Lactobacillus curvatus and Lactobacillus sakei and crossreacted with JPT57 in an HLA-DQ-dependent manner ( Fig. 6a ). Peptide-binding studies revealed that these three peptides bind with an intermediate binding affinity to HLA-DQ7 and HLA-DQ8 ( Fig. 6b,c ). Molecular models of these bacterial peptides in HLA-DQ8 illustrate the similarities with VCL-DERAA ( Fig. 6d–g , Supplementary Figs 19–21 ). 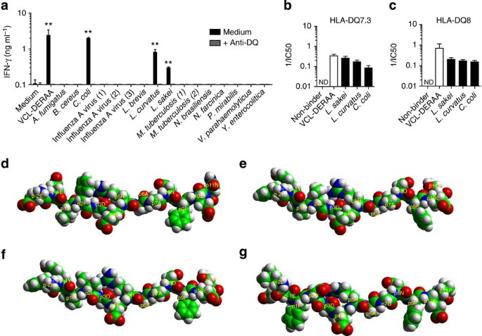Figure 6: TCR crossreactivity of vinculin and bacterial DERAA epitopes. (a) IFN-γ ELISA on supernatant of T cell clone JPT57 stimulated with HLA-DQ8-positive B-LCLs and alanine-substituted VCL-DERAA peptides. This experiment was performed three times, the plot shows a representative experiment. Two-sided statistical analysis was performed using a Student’st-test with * indicatingP<0.05 and ** indicatingP<0.001. (b,c) Competitive binding of HLA-DQ7.3 (b) and HLA-DQ8 (c) to a non-binding negative control peptide, an unbiotinylated positive control peptide and epitopes fromLactobacillus curvatus,Lactobacillus sakeiandCampylobacter coli. Binding experiments were performed three times. The error bars show the variation between the different experiments. (d–g) Side views of HLA-DQ8 complexed with the vinculin-DERAA peptide (d) and peptides derived fromLactobacillus curvatus(e),Lactobacillus sakei(f) andCampylobacter coli(g) in space-filling mode at pH 7.4 (extracellular), obtained by energy minimization as described in the methods section. Each peptide is shown in atomic colour code: oxygen, red; nitrogen, blue; hydrogen, white; carbon, green; sulfur, yellow. Error bars are s.e.m. Figure 6: TCR crossreactivity of vinculin and bacterial DERAA epitopes. ( a ) IFN-γ ELISA on supernatant of T cell clone JPT57 stimulated with HLA-DQ8-positive B-LCLs and alanine-substituted VCL-DERAA peptides. This experiment was performed three times, the plot shows a representative experiment. Two-sided statistical analysis was performed using a Student’s t -test with * indicating P <0.05 and ** indicating P <0.001. ( b , c ) Competitive binding of HLA-DQ7.3 ( b ) and HLA-DQ8 ( c ) to a non-binding negative control peptide, an unbiotinylated positive control peptide and epitopes from Lactobacillus curvatus , Lactobacillus sakei and Campylobacter coli . Binding experiments were performed three times. The error bars show the variation between the different experiments. ( d – g ) Side views of HLA-DQ8 complexed with the vinculin-DERAA peptide ( d ) and peptides derived from Lactobacillus curvatus ( e ), Lactobacillus sakei ( f ) and Campylobacter coli ( g ) in space-filling mode at pH 7.4 (extracellular), obtained by energy minimization as described in the methods section. Each peptide is shown in atomic colour code: oxygen, red; nitrogen, blue; hydrogen, white; carbon, green; sulfur, yellow. Error bars are s.e.m. Full size image Thus, these data show that the RA-susceptibility alleles HLA-DQ7 and HLA-DQ8 can present both VCL-DERAA and related microbe-derived epitopes to T cells and that such T cells can be crossreactive to vinculin and bacterial epitopes, thereby providing an explanation for the presence of activated self-reactive CD4 + T cells directed to vinculin in peripheral blood. The strong connection between the HLA locus and RA has been known for more than 35 years. The complex HLA class II associations and the diverse ACPA responses in RA patients suggest the presence of multiple aetiological pathways. To unravel these pathways, identifying the relevant autoantigens is crucial. We here present evidence favouring the involvement of vinculin in the emergence of ACPA + disease. This cytoskeletal protein was recently found to be citrullinated in vivo in the synovial fluid. We now show that it is recognized by ACPA as well, thereby adding it to a still selective list of targets. Moreover, we identified an epitope from vinculin recognized by CD4 + T cells restricted to HLA-DQ molecules predisposing to ACPA + RA. The core amino-acid sequence (DERAA) is also present in many pathogens and in HLA-DRB1*13, a molecule encoded by an HLA locus associated with protection against ACPA + RA. We have also shown that a single TCR can recognize both a vinculin-DERAA epitope as well as DERAA epitopes from microbes, indicating the crossreactive nature of ‘DERAA’-directed T cell responses. More importantly, such T cell responses appear absent from donors carrying HLA-DRB1*13 as DERAA-directed T cell responses to either pathogen- or vinculin-derived DERAA epitopes were lacking in these subjects. Even donors that harboured HLA-DRB1*13 next to predisposing HLA alleles were unable to respond to vinculin-DERAA. Together these data indicate a novel pathway that explains several of the protective and predisposing HLA-effects associated with ACPA + RA ( Fig. 7 ). In short, recognition of citrullinated vinculin by B cells will lead to the presentation of the ‘VCL-DERAA’ epitope in the context of HLA class II molecules. The HLA-DQ molecules genetically linked to the predisposing HLA-SE-molecules are particularly good in presenting DERAA-containing peptides. The DERAA-directed T cells primed against various pathogens harbouring DERAA-containing proteins cross-react with the VCL-DERAA peptide and provide help to the B cells, ultimately leading to a strong ACPA response. Subjects born with HLA-DRB1*13, will present the HLA-DRB1*13-derived DERAA-peptide in the thymus, leading to tolerization of the DERAA-reactive T cell response and hence the inability to provide help to ACPA-producing B cells via this pathway and thereby the emergence of ACPA + RA ( Fig. 7 ). 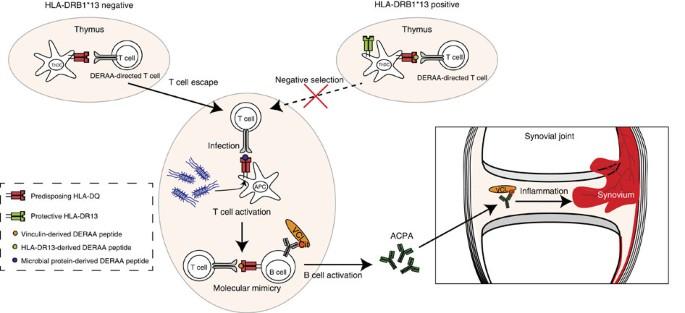Figure 7: Schematic representation of the proposed role of DERAA-directed CD4+T cells in ACPA+RA. DERAA-directed T cells are restricted to RA-predisposing HLA-DQ5, -DQ7.3 and –DQ8 molecules. In carriers of these HLA-DQ molecules, DERAA-directed T cells can become activated on contact with microbes. These activated T cells can subsequently crossreact with a DERAA epitope derived from vinculin resulting in the activation of citrulline-directed B cells and the production of ACPA directed to citrullinated vinculin or vinculin-linked proteins. Citrullinated vinculin is present in the synovial compartment and is a target of ACPA. Binding of ACPA to its target can induce antibody-mediated effector mechanisms thereby contributing to synovial inflammation. In HLA-DRB1*13-positive individuals, a HLA-DRB1*13-derived DERAA epitope is presented by predisposing HLA-DQ molecules to CD4+T cells resulting in their negative selection, thereby protecting against the development of ACPA+RA. Figure 7: Schematic representation of the proposed role of DERAA-directed CD4 + T cells in ACPA + RA. DERAA-directed T cells are restricted to RA-predisposing HLA-DQ5, -DQ7.3 and –DQ8 molecules. In carriers of these HLA-DQ molecules, DERAA-directed T cells can become activated on contact with microbes. These activated T cells can subsequently crossreact with a DERAA epitope derived from vinculin resulting in the activation of citrulline-directed B cells and the production of ACPA directed to citrullinated vinculin or vinculin-linked proteins. Citrullinated vinculin is present in the synovial compartment and is a target of ACPA. Binding of ACPA to its target can induce antibody-mediated effector mechanisms thereby contributing to synovial inflammation. In HLA-DRB1*13-positive individuals, a HLA-DRB1*13-derived DERAA epitope is presented by predisposing HLA-DQ molecules to CD4 + T cells resulting in their negative selection, thereby protecting against the development of ACPA + RA. Full size image The variation of HLA-DR and HLA-DQ molecules in the human population is enormous. We have shown that predisposing HLA-DQ molecules are particularly good at presenting the VCL-DERAA epitope. Interestingly, the absence of VCL-DERAA affinity for a wide variety of other tested HLA-DR or HLA-DQ molecules could indicate a selective presentation by these HLA risk molecules. Next to a role of predisposing haplotypes, we also focussed on the protective effect of HLA-DRB1*13 alleles. However, the DERAA sequence can also be found in other HLA-DRB1 alleles (*04:02, *11:02, *11:03), which are rare in Caucasian populations. These alleles have previously been implicated in protection from ACPA + RA, but their allele frequency hampers functional studies [30] , [31] , [32] . Interestingly, it has been previously reported that the processing of these alleles results in the generation of a similar HLA-DERAA epitope suggesting that these alleles could all protect via the pathway that we have described [22] . The place in time at which HLA-DR13 mediates protection from the development of ACPA and/or ACPA + disease, or its relation to epitope spreading of the ACPA response is currently not known and would be relevant to determine in future studies. Recent evidence showed that the ACPA response matures before disease onset and that the HLA system could be involved in this [13] , [33] . It is intriguing to speculate that infections such as by DERAA-containing microbes are involved in this expansion. Molecular mimicry of self-proteins with pathogenic proteins was proposed as a mechanism to break T cell tolerance, allowing the development of autoimmune disease [26] , [27] . Interestingly, the DERAA sequence is also present in proteins from many (common) microbes allowing priming of DERAA-directed T cells. In mouse models, it was shown that low-avidity T cells to tissue-restricted antigens can persist without signs of anergy and unresponsiveness. Infection lowers the threshold for T cell activation resulting in the induction of autoimmunity and memory formation [34] . Infection could also induce autoimmunity via molecular mimicry of microbial proteins with self-proteins. We now identified crossreactive epitopes from the gut-residing bacteria L. sakei , L. curvatus and C. coli . It was shown that acute gastrointestinal infections can induce loss of T cell tolerance to (commensal) gut microbes, resulting in the activation of microbiota-specific T cells, their differentiation to inflammatory effector cells and formation of memory T cells [35] . A recent study on the fecal microbiota of RA patients compared with controls demonstrated a significant increase in Lactobacillus species, together providing a rationale for a role of such bacterial species in the formation of DERAA-directed T cell responses [36] . Together our study provides a mechanistic clue on the HLA–RA connection, including both predisposing and protective HLA effect, and warrants further studies addressing the possibility to target DERAA-directed T cells in the prevention of ACPA + RA. Cells and sera HLA-typed buffy coats from healthy volunteers were obtained from the blood bank (Sanquin, The Netherlands). PBMCs and sera from RA patients were derived from patients participating in the Leiden Early Arthritis Clinic cohort [37] . All RA patients fulfilled the American College of Rheumatology (formerly the American Rheumatism Association) 1987 revised criteria for the classification of RA. A total of 178 RA patients were used in the current analyses. Patient samples were compared with 80 control samples from healthy individuals also living in the Leiden area. PBMCs were isolated using a standard Ficoll procedure. The protocols were approved by the Leiden University Medical Center ethics committee and informed consent was obtained. Peptides Peptides were synthesized according to standard Fmoc ( N -(9-fluorenyl)methoxycarbonyl) chemistry using a SyroII peptide synthesizer (MultiSynTech, Witten, Germany). The integrity of the peptides was checked using reverse-phase high-performance liquid chromatography and mass spectrometry. For vinculin ELISPOT experiments, HLA class II-binding studies and T cell activation studies 15-mer vinculin epitope VCL 622–636 (VCL-DERAA; REEVFDERAANFENH) was used. To determine the peptide-binding register, the VCL622–636 peptide was modified: Truncated on the N- or C terminus or alanine-/arginine-substituted at different positions. For ELISPOT assays against common pathogens, pathogenic peptides were used derived from measles virus (SSRASDERAAHLPTS), influenza A virus (VFEFSDERAANPIVP), human herpesvirus 7 (LAARADERAAFPDVG), Bordetella pertussis (SPNLTDERAAQAGVT), Staphylococcus aureus (QDMNDDERAALTMAM), Haemophilus influenzae (RFHGDDERAAKVYEN), Salmonella enteritidis (PLMMDDERAAKVYEN) and Propionibacterium acnes (EEVFTDERAARLSHV). For the generation of T cell lines, these eight pathogenic peptides were pooled. Cell lines The following Epstein–Barr virus-transformed lymphoblastoid B-cell lines were used: BSM (DRB1*04:01;DQA1*03:01;DQB1*03:02, IHW9032), BOLETH (DRB1*04:01;DQA1*03:01; DQB1*03:02, IHW9031), BM21 (DQA1*05:01;DQB1*03:01,, IHW9043), JSM (DQA1*03:02;DQB1*03:01), APD (DRB1*13:01;DQA1*01:03;DQB1*06:03,, IHW9291), BC34 (DRB1*13:02;DQA1*01:02;DQB1 *06:04), WT8 (DQA1*01:02;DQB1*06:02, IHW9017), KAS116 (DRB1*01:01;DQA1*01:02; DQB1*05:01,, IHW9003) and 721.82 (DR/DQ-negative) [38] . Cells were maintained in IMDM (Lonza) supplemented with 10% heat-inactivated fetal calf serum. JSM and BC34 cells are derived from healthy HLA-typed donors that were Epstein–Barr virus transformed. HLA class II competitive peptide-binding assay Peptide-binding assays were performed, as described previously [39] . In short, cell lysates from HLA class II homozygous B-lymphoblastoid cell lines were incubated on SPVL3- (anti-HLA-DQ) or B8.11.2- (anti-HLA-DR) coated (10 μg ml −1 ) FluoroNunc 96-well plates at 4° C overnight. Titration ranges of the tested peptides (0 to 300 μM) were mixed with a fixed concentration (0.6 μM) of biotinylated indicator peptide and added to the wells. Bound indicator peptide was detected using europium–streptavidin (Perkin Elmer, Boston, MA) and measured in a time-resolved fluorometer (PerkinElmer, Wallac Victor2). IC50 values were calculated based on the observed binding of the test peptide against the fixed concentration indicator peptide. The IC50 value depicts the concentration of test peptide required for a loss of 50% of the indicator peptide signal. Enzyme-linked immunosorbent spot assay PBMCs were incubated in 96-well Multiscreen HA plates (Millipore) precoated with 5 μg ml −1 anti-IFN-γ capture antibody (clone 1-D1K; Mabtech) at 5 × 10 5 cells per well and stimulated in X-VIVO medium (LONZA) with 5 μg ml −1 peptide or with a mix of recall antigens consisting of 0.75 Lf ml −1 tetanus toxoid (Netherlands Vaccine Institute), 0.5 μg ml −1 tuberculin purified protein derivative (Netherlands Vaccine Institute) and 0.005% Candida albicans (HAL allergy). After 24 h incubation at 37 °C, plates were extensively washed and incubated with 0.3 μg ml −1 biotin-labelled anti-IFN-γ detection antibody (clone 7-B6-1; Mabtech) for 2 h at RT, with 1,000 × diluted ExtrAvidin-Alkaline phosphatase (Sigma-Aldrich) for 1 h at RT and with 5-Bromo-4-chloro-3-indolyl phosphate/Nitro blue tetrazolium (Sigma-Aldrich). Spots were analysed using the BioSys Bioreader 3000pro. Circular spots with a size of 80–450 μm were included. Flow cytometry Polyclonal CD4 + T cell lines were generated by stimulating 3 × 10 6 PBMCs per well in a 24-well plate with 5 μg ml −1 peptide for 7 days in IMDM supplemented with 5% human serum (Sanquin). After 7 days, 1.5 × 10 6 autologous PBMCs per well were plated in 24-well plates for 2 h. After 2 h, non-adherent cells were removed and adherent cells were pulsed with 5 μg ml −1 peptide and used as feeders for 10 6 T cells. After 1 h, 10 μg ml −1 brefeldin A was added. Cells were incubated overnight and used for intracellular cytokine staining. The cells were incubated with fluorochrome-conjugated antibodies recognizing CD4, (Clone RPA-T4; BD biosciences), CD14 (Clone 61D3; eBioscience) and CD25 (Clone M-A251; BD biosciences), after which they were permeabilized using CytoFix CytoPerm Kit (BD Biosciences). After washing, cells were incubated with PE-labelled anti-IFN-γ or matching isotype control. Cells were taken up in 1% paraformaldehyde until flow cytometric acquisition. Flow cytometry was performed on FACS Calibur (BD biosciences) or LSR II (BD biosciences). Analysis was performed using FACS Diva (BD biosciences) and FlowJo software. T cell cloning JPT57 was generated from an HLA-DRB1*04:05/01:01;DQ8/DQ5 donor. PBMCs were cultured for 7 days in the presence of 10 μg ml −1 of VCL-DERAA peptide and restimulated with VCL-DERAA-pulsed antigen-presenting cells. After 1 week, cells were restimulated with 150 U ml −1 rIL-2. After two rounds of restimulation, T cell lines were tested for their specificity. The wells responding to VCL-DERAA peptide were cloned in a limiting dilution of 0.3 cells per well resulting in the isolation of clone JPT57. T cell clone D2C18 was generated from an HLA-DRB1*04:01;DQ2/DQ8-positive donor. CD4 + T cells and CD14 + monocytes were isolated from PBMCs using antibodies bound to magnetic beads from, respectively, Dynal and Miltenyi. CD4 + T cells were labelled with 1 μM CFSE (Invitrogen) and incubated in a 2:1 ratio with CD14 + monocytes with 30 μg ml −1 PathMix. After 6 days, CD3 pos CD4 pos CD25 pos CD14 neg DAPI neg CFSE low cells were sorted by FACS aria (BD). Isolated CD4 + T cells were rested in medium containing 20 IU ml −1 rIL-2 (Peprotech). After 3 days, the cells were cloned in a limiting dilution of 0.3 cells per well resulting in the isolation of CD4 + T cell clone D2C18. T cell activation To determine IFN-γ production by T cell clones in response to peptide stimulation, 50,000 T cells were incubated in a 1:1 ratio with B-LCL lines pulsed with 10 μg ml −1 of peptide for 3–6 h. After 3 days, the supernatant was collected and an IFN-γ ELISA (eBioscience) was used to determine the concentration of IFN-γ. For measurement of T cell proliferation, 50,000 T cells were incubated in a 1:1 ratio with radiated (3000RAD) autologous PBMCs pulsed with 10 μg ml −1 of peptide for 3–6 h in IMDM supplemented with 5% human serum. After 3 days, cells were cultured for 16–20 h with [ 3 H]thymidine (0.5 μCi per well). 3 H incorporation was measured by liquid scintillation counting (1450 MicroBeta TriLux; PerkinElmer). Blocking experiments were performed by preincubating antigen-presenting cells for 1 h with 20 μg ml −1 anti-DQ (SPVL3), anti-DR (B8.11.2) and anti-DP (B7.21) blocking antibodies. Detection of anti-citrullinated vinculin antibodies Citrullinated vinculin was generated by incubation of 50 μg vinculin protein (Sanbio) in a volume of 200 μl containing 0.1 M Tris-HCl pH 7.6, 0.15 M CaCl 2 , and 10 U PAD4 (Sigma) for 4 h at 37 °C. Unmodified vinculin protein was generated by incubation of vinculin with PAD4 without CaCl 2 . Citrullinated and unmodified vinculin were loaded onto 10% SDS–polyacrylamide gels and transferred onto blotting membranes. Blots were blocked, washed and incubated in 1:500 diluted serum overnight at 4 °C. The sera were either ACPA + or ACPA − as determined by ELISA. Blots were incubated with horseradish peroxidase-labelled rabbit anti-human IgG (Dako) and visualized with chemiluminescence (ECL, Amersham). To analyse reactivity to vinculin by a monoclonal ACPA (anti-cFIB1.1, citrullinated fibrinogen), vinculin- or citrullinated vinculin-coated Nunc plates were incubated with 0.2 μg ml −1 anti-cFIB1.1 for 2 h at room temperature [28] . Bound antibody was detected using horseradish peroxidase-labelled rabbit anti-human IgG (Dako) and visualized with ABTS. Peptide ELISA was performed as described previously using biotinylated peptides coated on streptavidin-precoated plates [40] . B-cell activation by JPT57 cells B cells were isolated from PBMCs of HLA-DQ8-positive healthy donors or ACPA-positive RA patients by magnetic anti-CD19-beads (Invitrogen). B cells were cultured in IMDM supplemented with 10% fetal calf serum, penicillin, streptomycin and glutamax. From healthy subjects, 30,000 B cells were co-cultured with different number of JPT57 cells in the presence of 5 μg ml −1 anti-IgM (JacksonImmunoresearch Laboratories) and with 10 μg ml −1 VCL-DERAA or 1 μg ml −1 PHA in round-bottom 96-well plates. After 7 days, IgG production by B cells was determined using a total IgG ELISA (Bethyl laboratories). From RA patients, 20,000 B cells were pulsed with 10 μg ml −1 VCL-DERAA peptide and co-cultured with 20,000 JPT57 cells in the presence of 5 μg ml −1 anti-IgM in round-bottom 96-well plates. After 7 days, ACPA production was determined by ELISA measuring reactivity against the CCP2-peptide in individual wells (EuroDiagnostica). Energy minimization Molecular simulations of HLA-DQ8(A1*0301/B1*302) and HLA–DQ7.3 (A1*0302/B1*0301) complexed with various peptides, experimentally shown to bind to these molecules, were carried out as previously described using the Discover Suite (programmes InsightII and Discover) of Accelrys (San Diego, CA, release of 2005) on a Silicon Graphics Fuel instrument, using a minimization approach previously described [41] , that is, 1,000 steps of the steepest gradient method, followed by 1,000 steps of the conjugate gradient method. Records of the energy of every step showed a continuous decrease in energy without any local minima and an energy asymptote for the last 300–400 steps of the conjugate gradient method. The base molecule was the crystal structure of HLA-DQ8 (A1*0301/B1*0302) with bound the insulin B11–23 peptide [42] . The region HLA-DQβ105-112 for which full coordinates were not available in the original data, was constructed by molecular replacement of the respective region from HLA-DR1 ( [43] ), after superposition of the β-plated sheet regions of the two molecules in the α1β1 domains. The binding registers of the vinculin and the bound microbial peptides were decided from the binding of truncated peptides as well as Arg-substituted peptides in presumed anchor positions; energy minimization of successive registers confirmed the registers predicted from the binding data. The rotamers for the peptide residues were chosen from a library of rotamers provided by the software database, to have no molecular clashes with the residues of HLA-DQ8. Minimizations were carried out either at pH 5.4 (endosomal pH) or 7.4 (extracellular). There are no similarly charged residues (for example, Glu–Glu) with their charged groups so close to each other as to require that one of the residues be uncharged. Occasionally runs were performed on a Silicon Graphics Octane instrument with previous releases of the same software with very similar results. Figures are drawn using the WebLabViewer v.3.5 and DSViewerPro software of Accelrys, the latter currently freely available on the web. In the figures a side view of the bound peptide with the eye level placed at the level of the peptide backbone and parallel to the HLA-DQ β-sheet floor is visualized with an atomic colour code as in the respective figure legend. In the Supplementary Figures , the α1β1 domains of the modelled HLA-DQ molecules in complex with given bound peptides are depicted in van der Waals surface representation, with colour and depiction conventions identical to those for the other figures. Several visible residues from the HLA-DQ molecule in contact with the antigenic peptide and potential contact with a cognate TCR in canonical orientation are shown in stick form with a transparent surface (atomic colour code: oxygen, red; nitrogen, blue; hydrogen, white; carbon, orange; sulfur, yellow). The antigenic peptide in the groove is shown in space filling form with the same atomic colour code as in Fig. 6d–g . Coordinates of all complexes shown in the various figures have been deposited in the Figshare repository under accession codes 1294716. MD simulations The simulated system consisted of the entire DQ8 molecule and the 13-residue peptide with the vinculin sequence Glu-Glu-Val-Phe-Asp-Glu-Arg-Ala-Ala-Asn-Phe-Glu-Asn. Titratable residues were assigned their most common ionization state at physiological pH, with the exception of DQ8 residue αGlu31, which was protonated. In the crystallographic structure of the DQ8:insulin complex, residues αGlu31 and βGlu86 are in direct contact [42] and their geometry and interactions with nearby residues and a crystallographic water suggest that at least one of them is protonated. A similar conclusion was reached for a pair of Glu and Asp residues in the pocket P6 of DR and I-E molecules [44] . We used the empirical model Propka [45] and a constant-pH Monte Carlo approach implemented in the program PROTEUS [46] to compute the pK of titratable groups in the crystallographic structure of HLA-DQ8, both in the absence and the presence of the peptides insulin and VCL-DERAA. Both methods agreed that the residues αGLU31 and βGLU86, near pocket P1, are strongly correlated; the predicted pKa values suggested that one of them should be protonated, most probably αGlu31. The initial coordinates of the protein heavy atoms were taken from the crystallographic structure of the DQ8:insulin complex (PDB accession code 1JK8) [42] . The peptide main chain heavy atoms were placed at the corresponding coordinates of the insulin main chain. Hydrogens were positioned by the HBUILD algorithm of the CHARMM programme [47] . The peptide side chain initial conformations were optimized with the program PROTEUS [45] . An additional control simulation studied the DQ8:insulin complex; for this system, the initial coordinates of the protein and peptide were taken from the corresponding crystallographic structure (PDB accession code 1JK8) [42] . The initial set-up of the simulation system was performed with the CHARMM-GUI interface [48] . A total of 70 crystallographic waters of the DQ8:insulin complex were retained. For the vinculin complex, crystallographic waters were minimized for 100 steps before the simulation, with the protein and peptide atoms kept fixed. The ligand complexes were immersed in a periodically replicated water box with the shape of a 117-Å truncated octahedron. Overlapping water molecules were omitted and 17 potassium anions were added (14 ions in the insulin complex), to neutralize the total charge. The final complex had 120,324 atoms (6,166 protein-ligand atoms); the insulin complex had 120,504 atoms (6,172 protein-ligand atoms). The simulations employed the molecular mechanics program CHARMM c37b2 (ref. 47 ). Protein atomic parameters were taken from the CHARMM36 all-atom force field with a CMAP backbone phi/psi energy correction [49] , [50] . Water parameters corresponded to the modified TIP3P water model [51] , [52] . Electrostatic interactions were calculated without truncation by the particle-mesh Ewald method [53] , with a parameter κ =0.34 for the charge screening, and sixth-order splines for the mesh interpolations. The Lennard–Jones interactions between atom pairs were switched to zero at a cutoff distance of 12 Å. The temperature was kept at T =300 K by a Nose–Hoover thermostat [54] with a mass of 2,000 kcal mol −1 ps −2 for the thermostat. The pressure was maintained at P =1 atm with a Langevin piston [55] , [56] . The piston mass was set to 1/20 of the total mass of the system and the collision frequency was set to 20 ps −1 . The classical equations of motion were solved by the leap-frog integrator. Bond lengths to hydrogen atoms and the internal water geometry were constrained to standard values via the SHAKE algorithm [57] , implemented into CHARMM. The structure was initially optimized by 100 energy minimization steps with the steepest-descent and adopted-basis Newton–Raphson algorithms. This was followed by an equilibration run, consisting of three 200-ps segments, in which the harmonic force constants were gradually lowered from 10 to 0 kcal mol −1 Å −2 . The production simulation had a duration of 3 ns (vinculin complex) and 4 ns (vinculin complex with ionized αGlu31 and insulin complex). A total of 300 and 400 snapshots were analysed for the vinculin- and insulin-DQ8 complex, respectively, extracted every 10 ps. All simulations were conducted with version c37b2 of the CHARMM programme [47] . Hydrogen bond occupancies and averaged intermolecular interaction energies were computed by in-house scripts. Molecular visualization was performed using the program VMD [58] . The interaction energies of selected peptide–protein residue pairs were computed by the following equation [59] , [60] : The first and second group of terms on the right-hand side of equation (1) describe, respectively, polar and non-polar interactions between R and R′; ‘Coul’ denotes Coulombic interaction, ‘GB’ denotes generalized born interaction, Δ S i is the change in the solvent accessible surface area of atom on binding and σ is a surface tension coefficient. The residue-pair interaction energies of equation (1) include solvent-mediated effects via the above GB and surface area terms. In the calculations of Supplementary Fig. 15 , R and R′ are distinct ligand and protein residues. We employed the GBSW Generalized Born model [61] , [62] , as implemented in the CHARMM programme. The coefficient σ was set to 0.005 kcal mol −1 Å 2 , for consistency with the GBSW parameterization. To compute the GB contributions, we removed all waters and ions from the simulation system and set the charge to zero for protein and peptide atoms other than those belonging to residues R and R′, respectively. The last term contains the difference in solvent accessible surface areas of groups R and R′ in the complex and unbound states. Coordinates of all complexes shown in the various figures have been deposited in the Figshare repository under accession code 1294716. Accession codes : The molecular models of DERAA peptides in complex with HLA-DQ molecules have been deposited in the Figshare repository under accession code 1294716 ( http://dx.doi.org/10.6084/m9.figshare.1294716 ). How to cite this article: van Heemst, J. et al. Crossreactivity to vinculin and microbes provides a molecular basis for HLA-based protection against rheumatoid arthritis. Nat. Commun. 6:6681 doi: 10.1038/ncomms7681 (2015).